Photo-enhanced antinodal conductivity in the pseudogap state of high-Tccuprates A major challenge in understanding the cuprate superconductors is to clarify the nature of the fundamental electronic correlations that lead to the pseudogap phenomenon. Here we use ultrashort light pulses to prepare a non-thermal distribution of excitations and capture novel properties that are hidden at equilibrium. Using a broadband (0.5–2 eV) probe, we are able to track the dynamics of the dielectric function and unveil an anomalous decrease in the scattering rate of the charge carriers in a pseudogap-like region of the temperature ( T ) and hole-doping ( p ) phase diagram. In this region, delimited by a well-defined T* neq ( p ) line, the photoexcitation process triggers the evolution of antinodal excitations from gapped (localized) to delocalized quasiparticles characterized by a longer lifetime. The novel concept of photo-enhanced antinodal conductivity is naturally explained within the single-band Hubbard model, in which the short-range Coulomb repulsion leads to a k -space differentiation between nodal quasiparticles and antinodal excitations. Superconductivity in the cuprates takes place when charge carriers are injected into a charge-transfer insulator [1] in which the carriers are localized by the strong electron–electron interactions. This surprising phenomenon has motivated a remarkable effort to understand to what extent the electron–electron interactions determine the physical properties of cuprates when tuning these materials away from the insulating state by increasing the hole concentration p and the temperature T . The physics of superconducting cuprates is further complicated by an anisotropic gap (pseudogap) in the electronic density of states (DOS), which opens well above the superconducting critical temperature ( T c ) at moderate doping and takes on maximal values close to the k =(± π ,0), (0,± π ) regions (antinodes) of the Brillouin zone (BZ) (ref. 2 ). In the same region of the p – T phase diagram, different ordered phases have been observed. Such phases can be favoured by the reduced kinetic energy of the carriers and might be associated with a quantum critical point underneath the superconducting dome T c ( p ) [3] , [4] . Indeed, a wealth of different broken symmetries, such as unusual q =0 magnetism [5] , [6] , [7] , charge-density waves (CDW) [8] , [9] , stripes [10] , nematic and smectic phases [11] , [12] , [13] , have been reported. The universal mechanism underlying the formation of the pseudogap continues to be the subject of intense research [14] , and the relation between the electronic interactions and the various ordering tendencies remains one of the major open questions. A possible scenario that reconciles this phenomenology is that the pseudogap emerges as an inherent effect of the strong short-range Coulomb repulsion, U , between two electrons occupying the same lattice site [15] . Considering the case of an isotropic Mott insulator, the U -driven suppression of charge fluctuations is expected to reduce the electron kinetic energy and render the electronic excitations increasingly localized in real space. Cluster generalization of dynamical mean-field theory (DMFT) calculations [16] , [17] , [18] suggests that the cuprates exhibit a similar U -driven reduction of kinetic energy that is, however, not uniform in momentum space. In the underdoped region, the antinodal excitations are indeed quasi-localized, with a T =0 divergent scattering rate that is reminiscent of the Mott insulator (see Fig. 1a ), whose self-energy (SE) diverges at low frequency and decreases at finite temperature. In contrast, the nodal (N) excitations in the vicinity of k =(± π /2,± π /2) still retain the essential nature of the quasiparticles (QPs) at large hole concentrations, that is, a scattering rate that increases when external energy is provided (see Fig. 1b ). The possible k -space differentiation between nodal QPs and antinodal excitations in the pseudogap phase has been hitherto elusive both to k -space-integrated equilibrium techniques, such as optical spectroscopy and resistivity measurements, that are mostly sensitive to the properties of nodal QPs and to conventional angle-resolved photoemission spectroscopy (ARPES), which has limits in capturing small temperature- and k -dependent variations of the electronic scattering rate. 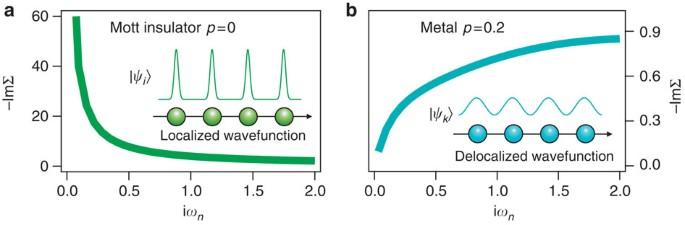Figure 1: Electron scattering rate of correlated systems. (a,b) The imaginary part of the electronic SE is calculated, as a function of the Matsubara frequencyωn=(2n+1)πkBT, by solving the single-band Hubbard model via single-site DMFT. The prototypical cases of the Mott insulator (p=0) and metallic system (p=0.2) are reported and contrasted. In the more realistic three-band Hubbard model, the same divergence of the SE is obtained as the charge-transfer insulating state is approached. Figure 1: Electron scattering rate of correlated systems. ( a , b ) The imaginary part of the electronic SE is calculated, as a function of the Matsubara frequency ω n =(2 n +1) πk B T , by solving the single-band Hubbard model via single-site DMFT. The prototypical cases of the Mott insulator ( p =0) and metallic system ( p =0.2) are reported and contrasted. In the more realistic three-band Hubbard model, the same divergence of the SE is obtained as the charge-transfer insulating state is approached. Full size image Here we adopt a non-equilibrium approach [19] based on ultrashort light pulses (≈100 fs) used to artificially prepare the system in a non-thermal state with an excess of antinodal (AN) excitations [20] . The key element of our experiment, which goes beyond single-colour pump-probe techniques [21] , [22] , [23] , is that the dynamics of the optical properties are simultaneously probed over an unprecedentedly broad energy range (0.5–2 eV). This technique allows us to probe the damping of the infrared reflectivity plasma edge and to directly relate the transient reflectivity variation, δ R ( ω , t ), to the instantaneous value of the optical scattering rate. From the outcome of time-resolved broadband spectroscopy, we infer that the transient non-thermal state created in the pseudogap phase is characterized by a scattering rate smaller than that at equilibrium. The emerging picture is that, on excitation, the localized antinodal states transiently evolve into more mobile states with a reduced scattering rate. This scenario is corroborated by DMFT calculations within the single-band Hubbard model and by time-resolved and ARPES (TR-ARPES) data in the pseudogap state. Finally, the generality of the concept of photo-enhanced antinodal conductivity in the pseudogap regime is demonstrated by combining the results obtained on different families of copper oxides (Bi- and Hg-based) in a single and universal phase diagram. Optical properties of cuprates Non-equilibrium optical spectroscopy is emerging as a very effective tool to unravel the different degrees of freedom coupled to electrons in correlated materials [19] , [24] . After the photoexcitation process, small variations of the equilibrium optical properties can be measured on a timescale faster than the recovery of the equilibrium QPs’ distribution, the complete restoration of the (long-range) orders [25] and the heating of the phonons [26] , thus unveiling an intriguing physics that cannot be accessed under equilibrium conditions. Single-colour time-resolved reflectivity measurements [21] , [22] , [23] have been applied in the past to study the pseudogap state, evidencing a characteristic dynamics proportional to the pseudogap amplitude (|Δ pg |) and a change of sign of the photoinduced reflectivity variation at T ≈ T *. Nonetheless, the inherent lack of spectral information of single-colour techniques precluded the understanding of the origin of this pseudogap-related reflectivity signal. Recent developments in ultrafast techniques now permit to overcome this limitation by probing the dynamics of the dielectric function over a broad frequency range. This paves the way to a quantitative modelling of the ultrafast optical response of the pseudogap phase. To properly model the dynamics of the optical properties measured in non-equilibrium conditions, we start by introducing the basic elements that characterize the equilibrium reflectivity, R eq ( ω ), of optimally doped Bi 2 Sr 2 Y 0.08 Ca 0.92 Cu 2 O 8+ δ (OP-YBi2212, hole-doping p =0.16, T c =96 K), shown in Fig. 2a . In the infrared region, the normal incidence R eq ( ω ) is dominated by a metallic-like response, which is characterized by a broad edge at the dressed plasma frequency ω p ≈1.25 eV. The infrared reflectivity of optimally and overdoped cuprates is well reproduced by the extended Drude model (EDM) [27] , [28] in which a frequency-dependent optical scattering time, τ ( ω , T ), accounts for all the processes that affect the QP lifetime, such as the electronic scattering with phonons, spin fluctuations or other bosons of electronic origin. 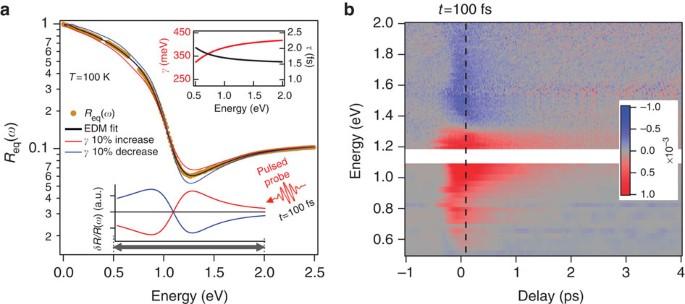Figure 2: Equilibrium and non-equilibrium optical spectroscopies. (a) The equilibrium reflectivity of an OP-YBi2212 sample, measured atT=100 K in the 0–2.5 eV spectral range, is reported (yellow dots). The black line is the fit of the equilibrium EDM to the data. The red (blue) curve is the reflectivity obtained from the EDM, in which an increase (decrease) in the optical scattering rate is artificially introduced. The bottom panel displays the relative reflectivity variation in the case of an increase (red line) and a decrease (blue line) in the optical scattering rate. The optical scattering rate,, is reported in the inset. The grey bar highlights the spectral range probed by the non-equilibrium spectroscopy. (b) The relative reflectivity variation, δR/R(ω,t), is reported as a function of the probe photon energy (ħω) and pump-probe delaytin the form of an intensity map. The colour coding for δR/R(ω,t) is indicated by the colourscale. Within the EDM, the optical scattering rate is connected to the single-particle SE by: Figure 2: Equilibrium and non-equilibrium optical spectroscopies. ( a ) The equilibrium reflectivity of an OP-YBi2212 sample, measured at T =100 K in the 0–2.5 eV spectral range, is reported (yellow dots). The black line is the fit of the equilibrium EDM to the data. The red (blue) curve is the reflectivity obtained from the EDM, in which an increase (decrease) in the optical scattering rate is artificially introduced. The bottom panel displays the relative reflectivity variation in the case of an increase (red line) and a decrease (blue line) in the optical scattering rate. The optical scattering rate, , is reported in the inset. The grey bar highlights the spectral range probed by the non-equilibrium spectroscopy. ( b ) The relative reflectivity variation, δ R / R ( ω , t ), is reported as a function of the probe photon energy ( ħω ) and pump-probe delay t in the form of an intensity map. The colour coding for δ R / R ( ω , t ) is indicated by the colourscale. Full size image where f is the Fermi–Dirac distribution and Σ( ζ , T ) and Σ*( ζ , T ) are the electron and hole k -space-averaged SEs. In Fig. 2a , we report the best fit of the EDM to the experimental R eq ( ω ) of OP-YBi2212 at T =100 K. In the calculation of the SE in equation (1), we use a recently developed model [29] , [30] , [31] that takes into account a non-constant QPs’ DOS, Ñ ( ω , T ), characterized by a pseudogap width Δ pg =40 meV (see Methods section). The k -space-integrated electronic DOS is recovered completely between Δ pg and 2Δ pg . The Ñ ( ω , T ) extracted by optical spectroscopy (see Methods; Supplementary Notes 1 and 2 ; Supplementary Figs 1 and 2 ) is in agreement with the outcome of tunnelling experiments [32] . The quality of the fit to the optical properties ( Fig. 2a ) demonstrates that the EDM with a non-constant DOS is a very effective tool to extract the scattering properties of the charge carriers, at least for moderate hole-doping concentrations. The possible failure of the EDM model is expected for hole-doping concentrations smaller than those of the samples studied in this work. The interband transitions at ħω >1.5 eV are accounted for by additional Lorentz oscillators at visible/ultraviolet frequencies. Focusing on the energy range that will be probed by the time-resolved experiment (0.5–2 eV), we note that τ ( ω ) has almost approached the asymptotic value τ ∞ ≈2 fs (see inset of Fig. 2a ). Therefore, we can safely assume that, in the 0.5–2 eV range, the damping of the reflectivity edge depends on the asymptotic value of the scattering rate, γ ∞ = ħ / τ ∞ . Non-equilibrium optical spectroscopy In the non-equilibrium optical spectroscopy, snapshots of the reflectivity edge of OP-YBi2212 are taken with 100 fs time resolution, as a function of the delay from the excitation with the 1.5 eV pump pulses. Considering that the temporal width of the probe pulses is much wider than the inherent scattering time of the charge carriers ( τ ∞ ≈2 fs), we can assume that the electronic excitations have completely lost any coherence on a timescale faster than the observation time. Therefore, the transient optical properties can be rationalized by changing some effective parameters in the equilibrium reflectivity. Notably, R eq ( ω , γ ∞ ) exhibits an isosbestic point (see Fig. 2a ) at the frequency . At this frequency, the reflectivity is independent of γ ∞ and, for small δ γ ∞ changes, it can be expanded as δ R ( ω , γ ∞ )=[∂ R(ω)/ ∂ γ ∞ ]δ γ ∞ , where [∂ R ( ω )/∂ γ ∞ ]>(<)0 for (see Supplementary Note 3 ; Supplementary Fig. 3 ). Therefore, the reflectivity variation, measured over a broad frequency range across , can provide a direct information about the instantaneous value of the total scattering rate during the thermalization process of the photoinduced non-equilibrium QP population. In the bottom panel of Fig. 2a , we report the normalized reflectivity variation δ R / R ( ω ), calculated from the equilibrium EDM model by assuming a positive (red line) or negative (blue line) variation of the total scattering rate, γ ∞ . The reflectivity variation associated with a change in γ ∞ extends over a broad frequency range and it changes sign when crossing the isosbestic point . Figure 2b shows the frequency-resolved measurements on OP-YBi2212 at T =100 K, as a function of the delay t from the pump pulse. The relative reflectivity variation δ R / R ( ω , t )=[ R neq ( ω , t )− R eq ( ω )]/ R eq ( ω ), where R neq is the non-equilibrium reflectivity, is reported as a two-dimensional (2D) plot. The colour scale represents the magnitude of δ R / R ( ω , t ) as a function of t and of the probe photon energy ħω . Soon after the excitation, δ R / R ( ω , t ) is positive below , whereas a negative signal is detected above . When compared with the δ R / R ( ω ) calculated for δ γ ∞ <0 (bottom panel of Fig. 2a ), the measured δ R / R ( ω , t ) suggests a transient decrease in the QP scattering rate soon after the excitation with the pump pulse. To substantiate the possible transient variation of γ ∞ , a differential model is used to quantitatively analyse the δ R / R ( ω , t ) signal. This approach consists in finding out the minimal set of parameters that should be changed in the equilibrium dielectric function to satisfactorily reproduce the measured δ R / R ( ω , t ) at a given time t . The main goal of this procedure is to disentangle the contributions of the genuine variation of γ ∞ , from that of possible photoinduced band-structure modifications, such as the transient filling of the pseudogapped electronic states [31] , [33] . In Fig. 3 , we report a slice of δ R / R ( ω , t ) (red dots) at fixed delay time, that is, t =100 fs. δ R / R ( ω , t =100 fs) is qualitatively reproduced, over the whole probed frequency range, by modifying only two parameters in the equilibrium EDM, that is, Ñ ( ω , T ) and γ ∞ . In contrast, no change in the interband transitions and in the plasma frequency is required. This demonstrates that, in the probed spectral range, the δ R / R ( ω ) signal is not significantly affected by the transient change in the electronic occupation at the pump energy scale or by other excitonic-like processes and that the density of the charge carriers is not significantly modified by the excitation process. Similarly, Fig. 3 also displays the contributions to the δ R / R ( ω , t =100 fs) signal, as arising from the variation of Ñ ( ω , T ) (green line) and γ ∞ (blue line), separately. The central result is that a negative γ ∞ variation is necessary to reproduce δ R / R ( ω , t =100 fs). δ γ ∞ <0 corresponds to a narrowing of the reflectivity plasma edge around the isosbestic point at (see Fig. 2a ), which is detected as a broad reflectivity variation changing from positive to negative when moving to high frequencies. Quantitatively, the relative variation δ γ ∞ / γ ∞ =−(1.2±0.4) × 10 −2 is extracted from the fitting procedure. For sake of clarity, we show in Fig. 3 the total δ R / R ( ω ) calculated (black dashed line) by constraining a positive δ γ ∞ / γ ∞ =+1.2 × 10 −2 variation (red dashed line). In this case, the main features of the measured δ R / R ( ω ) cannot be, even qualitatively, reproduced. This demonstrates that, while the experimental uncertainties can affect the absolute value of δ γ ∞ / γ ∞ , the transient photoinduced decrease in the scattering rate is a robust experimental fact that is unaffected by possible uncertainties, such as fluence fluctuations or changes in the pump-probe overlap. 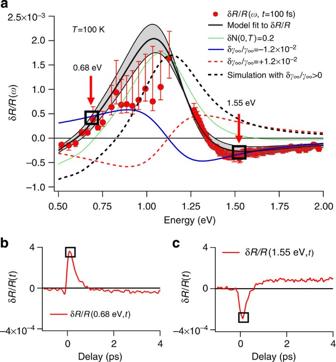Figure 3: Differential model for the non-equilibrium reflectivity. (a) The δR/R(ω,t=100 fs), measured on the OP-YBi2212 sample atT=100 K, is reported (red dots). The solid black line is the result of the fitting procedure of the differential model to δR/R(ω,t=100 fs), in which the DOSÑ(ω,T) (see Methods) andγ∞have been considered as free parameters. The contribution of each effect is shown separately: the green line represents the filling of the pseudogap DOS (δÑ≡Ñneq(0,T)–Ñeq(0,T)=0.2±0.02), in agreement with recent time-resolved ARPES results33; the blue line is related to the relative decrease ofγ∞. The dashed red line represents the δR/R(ω) due to an increase in the scattering rate. The dashed black line represents the calculation of δR/R(ω), assuming δÑ=0.2 and δγ∞/γ∞=+1.2 × 10−2. The red arrows highlight the probe energies at which the dynamics of the δγ∞/γ∞variation is investigated. The measurements atω<1.2 eV have been performed by tuning the probe wavelength through an optical parametric amplifier (see Methods). Therefore, each point atω<1.2 eV belongs to a different time-domain measurement in which the uncertainty in the absolute amplitude (reported as a red bar) is larger than that of the measurements in theω>1.2 eV frequency range. The error bars, accounting for the uncertainties in the pump fluence, size and spatial overlap with the probe beam, have been used as the weight for the fit. (b,c) Single-color time traces at photon energiesħω=0.68 and 1.55 eV. Figure 3: Differential model for the non-equilibrium reflectivity. ( a ) The δ R/R ( ω , t =100 fs), measured on the OP-YBi2212 sample at T =100 K, is reported (red dots). The solid black line is the result of the fitting procedure of the differential model to δ R/R ( ω , t =100 fs), in which the DOS Ñ ( ω , T ) (see Methods) and γ ∞ have been considered as free parameters. The contribution of each effect is shown separately: the green line represents the filling of the pseudogap DOS (δ Ñ ≡ Ñ neq (0, T )– Ñ eq (0,T)=0.2±0.02), in agreement with recent time-resolved ARPES results [33] ; the blue line is related to the relative decrease of γ ∞ . The dashed red line represents the δ R/R ( ω ) due to an increase in the scattering rate. The dashed black line represents the calculation of δ R/R ( ω ), assuming δ Ñ =0.2 and δ γ ∞ / γ ∞ =+1.2 × 10 −2 . The red arrows highlight the probe energies at which the dynamics of the δ γ ∞ / γ ∞ variation is investigated. The measurements at ω <1.2 eV have been performed by tuning the probe wavelength through an optical parametric amplifier (see Methods). Therefore, each point at ω <1.2 eV belongs to a different time-domain measurement in which the uncertainty in the absolute amplitude (reported as a red bar) is larger than that of the measurements in the ω >1.2 eV frequency range. The error bars, accounting for the uncertainties in the pump fluence, size and spatial overlap with the probe beam, have been used as the weight for the fit. ( b , c ) Single-color time traces at photon energies ħω =0.68 and 1.55 eV. Full size image The characteristic relaxation time ŧ of the measured δ γ ∞ is obtained by fitting the function δ R / R ( t )=δ R / R (0)exp(− t / ŧ ) to the time-resolved traces at fixed frequencies. In particular, we focus on the time traces at ħω =0.68 and 1.55 eV, shown in Fig. 3b,c , for which the contribution from the Ñ ( ω , T ) variation is negligible. The resulting value, ŧ =600±50 fs (see Supplementary Note 4 ; Supplementary Fig. 4 ), is of the same order as that of the time required for the complete heating of the lattice and for the recovery of the equilibrium QPs’ population, as will be shown by the time-resolved photoemission measurements. Interestingly, on the picosecond timescale, the δ R / R ( ω ) signal is qualitatively opposite to the signal at t ≈100 fs, as shown by the time traces in Fig. 3b,c . In particular, it changes from negative to positive as ω increases and crosses . The δ R / R ( ω , t >1 ps) signal can be reproduced by a broadening of the reflectivity edge, equivalent to an increase in the scattering rate (δ γ ∞ / γ ∞ =10 −4 ), with a negligible contribution from the variation of Ñ ( ω , T ). This γ ∞ increase is compatible with a local effective heating (δ T =0.6 K) of the lattice, which can be estimated considering the pump fluence (10 μJ cm −2 ) and the specific heat of the sample (see Supplementary Note 5 ; Supplementary Fig. 5 ). The transient decrease in the total electronic scattering rate, measured on the sub-picosecond timescale at T =100 K, is a novel finding that contrasts both with the results [26] obtained well above the pseudogap temperature and with the behaviour expected for a metallic system. In the latter case, the scattering rate should increase as energy is delivered, either adiabatically or impulsively. Furthermore, as inferred from the δ R / R ( ω , t ) measured in local quasi-equilibrium conditions ( t >1 ps), this anomalous δ γ ∞ <0 cannot originate from the partial quench of an order parameter or a temperature-induced decrease in the electron–boson coupling. In fact, the expected positive δ γ ∞ >0 is recovered at t >1 ps, although on this timescale an increase in the effective electronic and bosonic temperatures and the related amplitude decrease in the possible order parameter are attained. Non-equilibrium broadband optical spectroscopy crucially broadens the information that could be reached in the past by single-colour techniques. The quantitative modelling of the dynamics of the dielectric function in the 0.5–2 eV energy range demonstrates that, after the impulsive photoexcitation, the optimally doped YBi2212 sample at 100 K is driven into a non-equilibrium state, characterized by a scattering rate smaller than that at equilibrium (δ γ ∞ <0). In terms of the a.c. conductivity, this corresponds to a transient increase in the conductivity, once assumed a constant density of the charge carriers. The relaxation time of this photo-enhanced conductivity is ŧ =600±50 fs. On the picosecond timescale, the equilibrium distribution, dominated by nodal QPs, is recovered and a more conventional behaviour of the scattering rate (δ γ ∞ >0) is observed, in agreement with the outcomes of conventional equilibrium techniques, such as resistivity and optics [34] , [35] . The k -space-dependent non-equilibrium QP population Since the energy scale of the pump photons (1.5 eV) is much larger than the thermal ( k B T ≈10 meV) and the pseudogap (Δ pg ≈40 meV) energy scales, the photoinduced QPs’ distribution is expected to have no relation with the equilibrium one. The photoexcitation process can be roughly reduced to two main steps. In the first step, the pump pulse is absorbed creating electron–hole excitations extending from −1.5 to +1.5 eV across the Fermi energy ( E F ) and with a distribution that is regulated by the joint DOS of the photoexcitation process. In consequence of the extremely short scattering time of high-energy excitations ( τ ∞ = ħ/γ ∞ ≈2 fs), this photoexcited population undergoes a fast energy relaxation related to multiple scattering processes that lead to the creation of excitations at energies closer to E F . Considering the k -space-integrated DOS in the pseudogap state, a high density of excitations is expected to accumulate, within the pump-pulse duration (0–100 fs), in the Δ pg −2Δ pg energy range from E F . In the second and slower step, the subset of scattering processes that allow large momentum exchange, while preserving the energy conservation, leads to the recovery of a quasi-equilibrium distribution dominated by nodal QPs. Considering the phase-space constraints for these processes, the redistribution of excitations in the k -space is expected to be effective on the picosecond timescale. To directly investigate the k -space electron distribution after the photoexcitation process with 1.5 eV ultrashort pulses, we apply a momentum-resolved technique. TR-ARPES (see Methods section) is applied to measure the transient occupation at different k -vectors [36] , [37] along the Fermi arcs (see Fig. 4a ) of a Bi 2 Sr 2 CaCu 2 O 8+δ single crystal at T =100 K. When considering the TR-ARPES spectra at fixed angles Φ from the antinodal direction (see Fig. 4a ), the pump excitation results in a depletion of the filled states below E F and a filling of the states above E F [36] . In the following, we will focus on the integral ( I ) of the TR-ARPES spectra for E > E F , which is proportional to the total excess of excitations in the empty states. 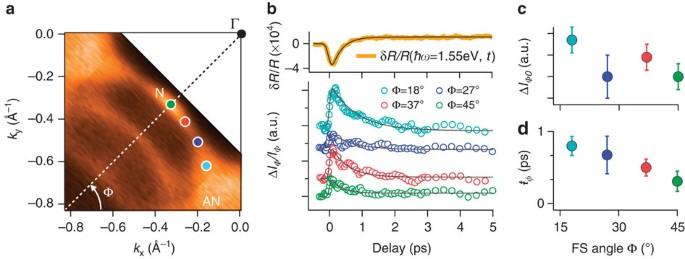Figure 4: Equilibrium and non-equilibrium photoemission. (a) The YBi2212 FS, measured by conventional ARPES at 100 K, is reported. The two FS replicas surrounding the main FS are due to surface reconstruction. The Γ point and the FSk-space regions where the TR-ARPES measurements have been performed are indicated by full dots. Φ is the FS angle from the antinode. (b) The normalized integrated variation of the TR-ARPES intensity aboveEF, ΔIΦ(t)/IΦ, is reported for different points along the Fermi arcs (Φ=18°, 27°, 37°, 45°). Solid lines are the fit to the data with a single exponential decay,. In the top panel, the δR/R(t) trace at 1.55 eV is reported for comparison. (c,d) The maximum intensity variation, ΔIΦ0, and the decay time,, of the non-equilibrium transient population measured by TR-ARPES are reported as a function of Φ. The error bars include the experimental uncertainty related to the possible alignment errors of the sample angle. Figure 4b reports the variation of I normalized to the intensity before the arrival of the pump pulse (Δ I Φ ( t )/ I Φ ) as a function of Φ. For each value of Φ, Δ I Φ ( t )/ I Φ is fitted by a single exponential decay of the form Δ I Φ0 exp(− t / ŧ Φ ), convoluted with a Gaussian function to account for the finite temporal resolution (~100 fs). Figure 4c,d shows the k -dependent values of Δ I Φ0 and ŧ Φ extracted from the fitting procedure. Within the error bars, Δ I Φ0 increases by a factor 3 when moving from the node (Φ=45°) towards the antinodal region of the BZ, indicating an effective photoinjection of AN excitations. This situation is dramatically different from that expected in equilibrium conditions, in which the number of excitations is governed solely by the Fermi–Dirac distribution at temperature T . In this case, the excitations’ density should significantly decrease when approaching the AN region of the BZ, as a consequence of the gap Δ pg >> k B T in the density of electronic states. Another notable result is that the relaxation time ŧ Φ is k -dependent, increasing from 300 to 800 fs when moving from the N to the AN region. These values are much larger than the total optical scattering time ( τ ∞ = ħ / γ ∞ ≈2 fs), which demonstrates that the recovery of a quasi-equilibrium QPs’ distribution is severely constrained, either by the phase space available for the scattering processes simultaneously conserving energy and momentum, or by some bottleneck effect related to the emission of gap-energy bosons during the relaxation of AN excitations. Figure 4: Equilibrium and non-equilibrium photoemission. ( a ) The YBi2212 FS, measured by conventional ARPES at 100 K, is reported. The two FS replicas surrounding the main FS are due to surface reconstruction. The Γ point and the FS k -space regions where the TR-ARPES measurements have been performed are indicated by full dots. Φ is the FS angle from the antinode. ( b ) The normalized integrated variation of the TR-ARPES intensity above E F , Δ I Φ ( t )/ I Φ , is reported for different points along the Fermi arcs (Φ=18°, 27°, 37°, 45°). Solid lines are the fit to the data with a single exponential decay, . In the top panel, the δ R / R ( t ) trace at 1.55 eV is reported for comparison. ( c , d ) The maximum intensity variation, Δ I Φ0 , and the decay time, , of the non-equilibrium transient population measured by TR-ARPES are reported as a function of Φ. The error bars include the experimental uncertainty related to the possible alignment errors of the sample angle. Full size image TR-ARPES demonstrates that, soon after the excitation with 1.5 eV pump pulses, an excess number of low-energy electron excitations is accumulated in the antinodal region. Furthermore, the relaxation time of this non-equilibrium distribution is significantly k -dependent. Taken together, these results prove that this non-equilibrium electron distribution in the k -space cannot be described by a Fermi–Dirac distribution with a single effective electronic temperature that is evolving in time. At the simplest level, we can assume that the effective temperature increase in the excitations in the antinodal region is larger than that of the nodal QP population. Notably, the k -space-averaged relaxation time of the non-equilibrium distribution, 〈 ŧ Φ 〉=550±200 fs, is the same, within the error bars, as of the relaxation time of the transient δ γ ∞ <0 measured by non-equilibrium optical spectroscopy. This result demonstrates the direct relation between the creation of a non-thermal distribution with an excess of antinodal excitations and the transient decrease in the scattering rate measured by non-equilibrium optical spectroscopy. T * neq ( p ) line emerging from non-equilibrium spectroscopy The use of ultrashort light pulses to manipulate the equilibrium QP distribution is crucial to investigate the cuprate phase diagram from a perspective that was hitherto inaccessible. In this section, we report on the T * neq ( p ) temperature below which the transient reduction of γ ∞ is observed via non-equilibrium optical spectroscopy. As shown in Fig. 3a , for ω significantly above ω p , the contribution to δ R / R ( ω , t ) due to the modification of Ñ ( ω ) is negligible. Therefore, single-colour pump-probe measurements at 1.55 eV probe photon energy contain the direct signature of the transient δ γ ∞ <0, in the form of a negative component [21] , [22] with relaxation time ŧ =600 fs [23] . 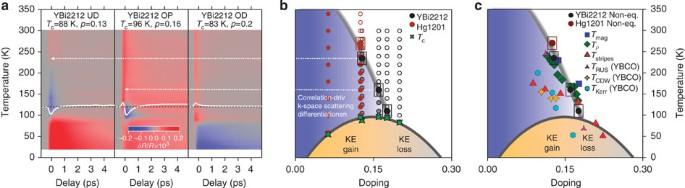Figure 5: The cuprate phase diagram from non-equilibrium spectroscopy. (a) The relative reflectivity variation δR/R(t) measured at the probe energy of 1.55 eV is reported as a function of the temperature (from 300 to 20 K) for three YBi2212 samples with different hole concentrations: underdoped (UD,Tc=88 K), optimally doped (OP,Tc=96 K) and overdoped (OD,Tc=83 K). The white lines are the δR/R(t) time traces at 110 K. (b) The general phase diagram of cuprates, as unveiled by non-equilibrium reflectivity measurements, is sketched. The pseudogap boundaryT*neq(grey curve) is determined reporting the temperature at which a negative component in the δR/R(t) signal appears on YBi2212 (black dots) and underdoped Hg1201 (purple dots) samples withTc=55 and 95 K. The grey circles indicate some of the temperatures at which the δR/R(t) data have been taken. The empty (full) circles correspond to a (non) zero negative signal in the δR/R(t) time traces. The green markers denote the critical temperatureTcof the samples. (c) TheT*neq(p) temperatures extracted from time-resolved optical spectroscopy experiments are compared with the values ofT*(p) extracted from resistivity45(green diamonds) and ultrasound spectroscopy14(purple stars) on Bi2212 and YBCO and with the onset of the newly-discoveredq=0 exotic magnetic order7,44(blue squares) on Bi2212 and Hg1201. We also compareT*neq(p) with the onset of ordered states, like CDW order47(yellow diamonds) in YBCO, fluctuating stripes48(red triangles) in Bi2212 and time-reversal symmetry-breaking states in YBCO46(blue hexagons). KE, kinetic energy; non-eq., non-equilibrium. Figure 5a reports some of the single-colour time traces measured as a function of the temperature (from 300 to 20 K) for different hole concentrations. The negative component (blue colour) appears in the δ R / R ( t ) signal at T * neq =240±20 K for p =0.13 and at T * neq =165±20 K for p =0.16. Above p =0.18, this negative δ R / R ( t ) signal is never detected on cooling the sample down to T c (see Supplementary Notes 6 and 7 ; Supplementary Figs 6, 7 and 8 ). A similar behaviour is also found for underdoped HgBa 2 CuO 4+δ (Hg1201; see Supplementary Note 8 ; Supplementary Figs 9,10 and 11 ). Hg1201 is considered a nearly ideal single-layer cuprate and exhibits a maximal critical temperature close to that of double-layer YBi2212 [38] , [39] . Collecting the results for the two materials on the same plot, we obtain a phase diagram that shows a universal behaviour for the properties of different copper-oxide-based superconductors having the same maximal critical temperature. Figure 5b shows that the p – T phase diagram of cuprates is dominated by an ubiquitous and sharp T * neq ( p ) boundary. Below this line, the pump-induced non-thermal distribution of the charge carriers exhibits a scattering rate smaller than that at equilibrium. This pseudogap-like T * neq ( p ) boundary meets the superconducting dome slightly above P =0.18. Below T c , the continuation of the T * neq ( p ) line delimits two regions of the superconducting dome that exhibit opposite variation of the optical spectral weight of intra- and inter-band transitions [24] , [40] , [41] , [42] , related to the crossing from a kinetic energy gain- to a potential energy gain-driven superconducting transition, consistent with predictions for the 2D Hubbard model [43] . Figure 5: The cuprate phase diagram from non-equilibrium spectroscopy. ( a ) The relative reflectivity variation δ R / R ( t ) measured at the probe energy of 1.55 eV is reported as a function of the temperature (from 300 to 20 K) for three YBi2212 samples with different hole concentrations: underdoped (UD, T c =88 K), optimally doped (OP, T c =96 K) and overdoped (OD, T c =83 K). The white lines are the δ R / R ( t ) time traces at 110 K. ( b ) The general phase diagram of cuprates, as unveiled by non-equilibrium reflectivity measurements, is sketched. The pseudogap boundary T * neq (grey curve) is determined reporting the temperature at which a negative component in the δ R / R ( t ) signal appears on YBi2212 (black dots) and underdoped Hg1201 (purple dots) samples with T c =55 and 95 K. The grey circles indicate some of the temperatures at which the δ R / R ( t ) data have been taken. The empty (full) circles correspond to a (non) zero negative signal in the δ R / R ( t ) time traces. The green markers denote the critical temperature T c of the samples. ( c ) The T * neq ( p ) temperatures extracted from time-resolved optical spectroscopy experiments are compared with the values of T *( p ) extracted from resistivity [45] (green diamonds) and ultrasound spectroscopy [14] (purple stars) on Bi2212 and YBCO and with the onset of the newly-discovered q =0 exotic magnetic order [7] , [44] (blue squares) on Bi2212 and Hg1201. We also compare T * neq ( p ) with the onset of ordered states, like CDW order [47] (yellow diamonds) in YBCO, fluctuating stripes [48] (red triangles) in Bi2212 and time-reversal symmetry-breaking states in YBCO [46] (blue hexagons). KE, kinetic energy; non-eq., non-equilibrium. Full size image Further insight into the T * neq ( p ) line unveiled by non-equilibrium optical spectroscopy is provided by the comparison with the pseudogap temperature T *( p ) estimated from complementary equilibrium techniques [7] , [14] , [44] , [45] (elastic neutron scattering, resistivity and resonant ultrasound spectroscopy) and with the onset temperature of different ordered states [46] , [47] , [48] (CDW, time-reversal symmetry-breaking states and fluctuating stripes). The picture sketched in Fig. 5c compares the main phenomenology on the most common materials with similar critical temperatures (Bi2212, Hg1201, YBCO). Remarkably, the T * neq ( p ) line almost exactly coincides with the pseudogap line estimated by resistivity measurements [45] and ultrasound spectroscopy [14] and with the onset of the newly-discovered q =0 exotic magnetic order [7] , [44] . The appearance of ordered states at T < T * is likely the consequence of the instability of the correlated pseudogap ground state on further cooling. The antinodal scattering rate The results reported in the previous sections suggest that the T * neq ( p ) line delimits a region in which the AN states evolve into more metallic ones (δ γ ∞ <0) on photoexcitation with the pump pulses. The generality of the results obtained calls for a general model that accounts for the phase diagram unveiled by the non-equilibrium optical spectroscopy. Considering that the measured transient decrease in the carrier scattering rate is faster than the complete heating of the lattice, we focus on the minimal model that neglects electron–phonon coupling and retains the genuine physics of correlations, that is, the 2D Hubbard Hamiltonian [49] , [50] . To compute the temperature-dependent SE in different positions of the BZ, we use the dynamical cluster approximation, a cluster extension of DMFT that captures the k -space differentiation of the electronic properties [17] between different regions of the BZ (see Methods section). Furthermore, long-range correlations are neglected to focus on the intrinsic effect of short-range correlations inside the chosen four-site cluster (see Methods section). At this stage, the increase in energy related to the pump excitation is mimicked by selectively increasing the effective temperature of the nodal and antinodal SEs. The FS of a lightly doped system is reported in Fig. 6a and exhibits a progressive smearing when moving from the nodes to the antinodes. This result is qualitatively in agreement with the FS experimentally measured by conventional ARPES in prototypical cuprates (compared with the ARPES data on optimally doped Bi 2 Sr 2 Y 0.08 Ca 0.92 Cu 2 O 8+ δ at 100 K reported in Fig. 4a ). The smearing of the FS at antinodes reflects a strong dichotomy between the scattering rate of nodal and antinodal excitations that can be captured by plotting the imaginary parts of the calculated SE, that is, the inverse QP lifetime, as a function of the effective temperature (see Fig. 6c ). In contrast to nodal QPs, whose scattering rate increases with temperature, the scattering rate of antinodal excitations exhibits a completely different evolution, decreasing as the effective temperature rises. This anomalous behaviour is related to the localized and gapped character of the antinodal fundamental excitations that experience very strong electronic interactions at low temperatures. The concept of delocalized QPs, characterized by a smaller scattering rate, is progressively recovered when the temperature increases. This striking dichotomy of the nature of the elementary excitations in the k -space is the consequence of a momentum-space selective opening of a correlation-driven gap, which eventually evolves into the full Mott gap at p =0. The same physics has been previously identified in calculations based on similar approaches (also using larger clusters to achieve a better momentum resolution) [16] , [17] , [18] , [51] . When the hole doping is increased (see Fig. 6b,d ), the k -space differentiation of N–AN fundamental excitations is washed out and a more conventional metallic behaviour is recovered. In this case, the delocalized QPs exhibit a gapless energy spectrum and a scattering rate that is proportional to a power function of the temperature over the entire BZ. 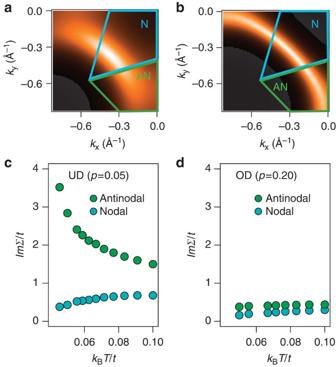Figure 6: The single-band Hubbard model and cluster-DMFT (CDMFT). (a,b) The FS reconstructed from CDMFT, for an UD (p=0.05) and an OD (p=0.2) sample, are reported. (c,d) The imaginary parts of the electronic SE, calculated through CDMFT as a function of the temperature, are reported for the UD and the OD samples, respectively. The effective temperature is expressed in units of the nearest-neighbor hoppingt. Assuming a reasonable valuet=0.3 eV,kT/t=0.1 corresponds toT=350 K. The values of the parameters used in the calculations areU=9tandt’=−0.25t. The imaginary parts of the SEs are calculated using dynamical cluster approximation (see ref.4and Methods section) and four equal-area partitions of the BZ. Following ref.4, the nodal and antinodal SEs are calculated in the regions centred ink=(0,0) (N) andk=(±π,0), (0,±π) (AN), as shown inaandb. Figure 6: The single-band Hubbard model and cluster-DMFT (CDMFT). ( a , b ) The FS reconstructed from CDMFT, for an UD ( p =0.05) and an OD ( p =0.2) sample, are reported. ( c , d ) The imaginary parts of the electronic SE, calculated through CDMFT as a function of the temperature, are reported for the UD and the OD samples, respectively. The effective temperature is expressed in units of the nearest-neighbor hopping t . Assuming a reasonable value t =0.3 eV, kT / t =0.1 corresponds to T =350 K. The values of the parameters used in the calculations are U =9 t and t ’=−0.25 t . The imaginary parts of the SEs are calculated using dynamical cluster approximation (see ref. 4 and Methods section) and four equal-area partitions of the BZ. Following ref. 4 , the nodal and antinodal SEs are calculated in the regions centred in k =(0,0) (N) and k =(± π ,0), (0,± π ) (AN), as shown in a and b . Full size image DMFT calculations thus confirm an intrinsic U -driven momentum-space differentiation of the electronic properties of cuprates at finite hole concentrations and temperatures. The nature of the AN states is similar to that of a Mott insulator in the sense that the scattering rate of AN states decreases when the internal energy of the system is increased. Wrapping up the experimental outcomes collected in this work, we can gain a novel insight into the pseudogap physics of high-T c cuprates. Time-resolved optical spectroscopy demonstrates that, on excitation with 1.5 eV pump pulses, the optical properties of cuprates transiently evolve into those of a more conductive system (δ γ ∞ <0). TR-ARPES shows that the k -space distribution of the electron excitations created by the pump pulse is characterized by an excess of AN electrons. Finally, the reported observation of a transient enhancement of the conductivity unveils a universal and sharp pseudogap-like T * neq ( p ) boundary in the p – T phase diagram. All these results cannot be rationalized in terms of the simple consequence of an anisotropic scattering of QPs with bosonic fluctuations, such as antiferromagnetic spin fluctuations. Although antiferromagnetic correlations may strongly influence the dynamics of AN excitations, the energy provided by the pump pulse should necessarily result in an increase in the boson density, leading to an increase in the scattering rate for all the timescales. Furthermore, the transient decrease in the scattering rate on the sub-picosecond timescale cannot be related to the presence of incipient charge orders, such as CDW, which are quenched by the pump pulse. The picosecond dynamics of conventional CDW has been widely studied in weakly correlated ( U ≈0) materials [25] , [52] . After the impulsive excitation, the characteristic timescale for the CDW recovery is on the order of several picoseconds, that is, much longer than the transient δ γ ∞ <0 measured in our work. Even assuming a purely electronic (and faster) density wave mechanism in cuprates, the photoinduced decrease in the scattering rate should monotonically decrease eventually approaching a zero value. This is in contrast with the experimental observation of a transition from δ γ ∞ <0 to δ γ ∞ >0 on the picosecond timescale. On the other hand, the Hubbard model provides a minimal framework for the interpretation of the pseudogap region of cuprates as unveiled by time-resolved spectroscopies. The pump pulse provides energy to the system in a non-thermal way, which can be schematized as a larger increase in the effective temperature of AN excitations as compared with that of nodal QPs. The transient decrease in the scattering rate (δ γ ∞ <0) is thus related to the evolution of AN excitations from Mott-like gapped excitations to delocalized QPs with a longer lifetime. On the picosecond timescale, the equilibrium electronic distribution is recovered and the expected δ γ ∞ >0 is measured. Although this picture does not exhaust all the properties of the pseudogap, it captures a key element of the universal and fundamental nature of the antinodal states, providing a backbone for more realistic multi-band descriptions [3] that could give rise to a broken-symmetry state originating from a quantum phase transition [4] at T =0. Furthermore, the short-range Coulomb repulsion induces a suppression of the charge fluctuations below the T * neq ( p ) line that is opposite to the effect of temperature. Therefore, the region of the cuprate phase diagram delimited by T * neq ( p ) is intrinsically prone to bulk [53] , [54] and surface [55] , [56] phase-separated instabilities, whose nature depends on the details of the Fermi surface (FS) of the particular system considered. Interestingly, the region of the cuprate phase diagram in which the optical photoexcitation creates a non-equilibrium state with longer lifetime closely corresponds to that in which the possibility of creating a transient superconductive state by tetrahertz excitation has been recently discussed [57] , [58] . These findings suggest a general tendency of copper oxides to develop, when photoexcited, a transient non-equilibrium state that is more conductive than the equilibrium phase. Samples The Y-substituted Bi2212 single crystals were grown in an image furnace by the travelling solvent floating-zone technique with a non-zero Y content to maximize T c [38] . The underdoped samples were annealed at 550 °C for 12 days in a vacuum-sealed glass ampoule with copper metal inside. The overdoped samples were annealed in a quartz test tube under pure oxygen flow at 500 °C for 7 days. To avoid damage of the surfaces, the crystals were embedded in Bi 2 Sr 2 CaCu 2 O 8+ δ powder during the annealing procedure. In both cases, the quartz tube was quenched into ice-water bath after annealing to preserve the oxygen content at annealing temperature. The Hg1201 single crystals were grown using a flux method, characterized and heat treated to the desired doping level [39] . The crystal surface is oriented along the ab -plane with a dimension of about 1 mm 2 . Hg1201 samples are hygroscopic. Therefore, the last stage of the preparation of the sample surface is done under a continuous flow of nitrogen, on which the sample is transferred to the high-vacuum chamber (10 −7 mbar) of the cryostat within a few minutes. Before each measurement, the surface is carefully checked for any evidence of oxidation. Optical spectroscopy The ab -plane dielectric function at equilibrium of the YBi2212 samples has been measured using conventional spectroscopic ellipsometry [59] . The dielectric function has been obtained by applying the Kramers–Kronig relations to the reflectivity for 50< ω /2 πc <6,000 cm −1 and directly from ellipsometry for 1,500< ω /2 πc <36,000 cm −1 . The δ R / R ( ω , t ) data presented in Fig. 2 have been acquired combining two complementary techniques [60] : (i) a pump supercontinuum-probe setup [61] , based on the white light generated in a photonic crystal fibre seeded by a Ti:sapphire cavity-dumped oscillator, to explore the visible–near infrared range of the spectrum (1.1–2 eV); (ii) a pump tunable-probe setup, based on an optical parametric amplifier seeded by a regenerative amplifier, to extend measurements in the infrared spectral region (0.5–1.1 eV). In both cases, the laser systems operate at 250 kHz repetition rate. The pump fluence is set to 10±2 μJ cm −2 for spectroscopic measurements. Single-colour measurements ( ħω =1.55 eV), presented in Fig. 5 , have been performed directly using the output of a cavity-dumped Ti:sapphire oscillator. The high-frequency modulation of the pump beam, combined with a fast scan of the pump-probe delay and lock-in acquisition, ensures a high signal-to-noise ratio (~10 6 ) and fast acquisition times, necessary to study the evolution of the time-resolved optical properties as a function of the temperature. Single-colour measurements have been performed with a pump fluence ranging from 3 to 30 μJ cm −2 . In all experiments, the pump photon energy is 1.55 eV. Samples are mounted on the cold finger of a closed-cycle cryostat. The temperature of the sample is stabilized within ±0.5 K. The EDM with a non-constant DOS In the EDM, the scattering processes are effectively accounted for by a temperature- and frequency-dependent scattering rate γ ( ω , T ), which is often expressed through the so-called memory function, M ( ω , T ). The dielectric function resulting from the EDM is: In the conventional formulation of the EDM (for more details, see refs 28 , 31 ), the calculation of the SE Σ( ω , T ) is based on the assumption of a constant DOS at the Fermi level. This approximation is valid at T =300 K in optimally and overdoped systems, but fails as the temperature and the doping decrease and a pseudogap opens in the electronic DOS. A further evolution of the EDM, accounting for a non-constant electronic DOS, has been recently developed [29] , and has been used to analyse spectroscopic data at equilibrium [30] . Within this model, the imaginary part of the electronic SE is given by: where n and f are the Bose–Einstein and Fermi–Dirac distribution functions, respectively; π(Ω) is the Bosonic function; and Ñ ( ω , T ) is the normalized DOS. The real part of the SE, Σ 1 ( ω , T ), can be calculated by using the Kramers–Kronig relations. The normalized DOS Ñ ( ω , T ) is modelled by [30] : Where Δ pg represents the (pseudo)gap width, while the normalized DOS at E F , that is, Ñ (0, T ), represents the gap filling. The π(Ω) function is extracted by fitting the EDM to the normal state optical properties [26] . π(Ω) is characterized by a low-energy part (up to 40 meV), a peak centred at ~60 meV and a broad continuum extending up to 350 meV. The analysis of the time- and frequency-resolved data is performed by modelling the non-equilibrium dielectric function ( ε neq ( ω )) and calculating the reflectivity variation through the expression: δ R/R ( ω , t )=[ R neq ( ω ,t)− R eq ( ω )]/ R eq ( ω ), where the normal incidence reflectivities are calculated as: R eq ( ω )=|[1−√ ε eq ( ω )]/[1+√ ε eq ( ω )]| 2 and R neq ( ω )=|[1−√ ε neq ( ω )]/[1+√ ε neq ( ω )]| 2 . The role of the finite penetration depth of the pump pulse ( d pu =160 nm @ 1.55 eV) is accounted for by numerically calculating δ R/R ( ω ) through a transfer matrix method, when a graded index of the variation of the refractive index n with exponential profile along the direction z perpendicular to the surface, that is, δ n =δ n 0 exp(− z / d pu ), is assumed. Photoemission spectroscopy The FS of YBi2212 reported in Fig. 4a has been measured by ARPES in equilibrium conditions. ARPES has been performed with 21.2 eV linearly polarized photons (He-α line from a SPECS UVS300 monochromatized lamp) and a SPECS Phoibos 150 hemispherical analyzer. Energy and angular resolutions were set to 30 meV and 0.2°. The Bi2212 samples studied by TR-ARPES are nearly optimally doped single crystals with a transition temperature T c =88 K. The samples have been excited by 55 fs laser pulses with a photon energy of 1.55 eV at 300 kHz repetition rate, at an absorbed fluence of 35 μJ cm −2 . The transient electron distribution was probed by time-delayed 80 fs, 6 eV laser pulses, photoemitting electrons, which were detected by a time-of-flight spectrometer. The energy resolution was 50 meV, the momentum resolution 0.05 Å −1 and the time resolution <100 fs. Cluster-DMFT and the Hubbard model The Hubbard Hamiltonian [49] , [50] is given by: where creates (annihilates) an electron with spin σ on the i ( j ) site, is the number operator, t ij the hopping amplitude to nearest and next-nearest neighbours, U the Coulomb repulsion between two electrons occupying the same lattice site and μ is the chemical potential that controls the total number of electrons in the N sites. The Hubbard model has been studied by means of a Cluster-DMFT that maps the full lattice model onto a finite small cluster (here a four-site cluster) embedded in an effective medium that is self-consistently determined as in standard mean-field theory. The method therefore fully accounts for the short-range quantum correlations inside the cluster. It has been shown by various authors that different implementations of this approach provide qualitatively similar results and reproduce the main features of the phase diagram of the cuprates, including the d-wave superconducting state and the pseudogap region that we discuss in the present paper. The calculations of this paper use the dynamical cluster approximation [62] prescription and the 4* patching of the BZ introduced in [17] and have been performed using finite-temperature exact diagonalization [63] to solve the self-consistent cluster problem using eight energy levels in the bath as in several previous calculations. The finite-temperature version of the exact diagonalization has been implemented as discussed in ref. 17 including typically 40 states in the low-temperature expansion of the observables. How to cite this article: Cilento, F. et al . Photo-enhanced antinodal conductivity in the pseudogap state of high-Tc cuprates. Nat. Commun. 5:4353 doi: 10.1038/ncomms5353 (2014).